Tonic inhibition in dentate gyrus impairs long-term potentiation and memory in an Alzheimer’s disease model Amyloid plaques and tau tangles are common pathological hallmarks for Alzheimer’s disease (AD); however, reducing Aβ production failed to relieve the symptoms of AD patients. Here we report a high GABA (γ-aminobutyric acid) content in reactive astrocytes in the dentate gyrus (DG) of a mouse model for AD (5xFAD) that results in increased tonic inhibition and memory deficit. We also confirm in human AD patient brains that dentate astrocytes have a high GABA content, suggesting that high astrocytic GABA level may be a novel biomarker and a potential diagnostic tool for AD. The excessive GABA in 5xFAD astrocytes is released through an astrocyte-specific GABA transporter GAT3/4, and significantly enhances tonic GABA inhibition in dentate granule cells. Importantly, reducing tonic inhibition in 5xFAD mice rescues the impairment of long-term potentiation (LTP) and memory deficit. Thus, reducing tonic GABA inhibition in the DG may lead to a novel therapy for AD. Alzheimer’s disease (AD) is a progressive neurodegenerative disorder with increasing morbidity among aging populations worldwide. Amyloid β peptide (Aβ) deposits and tau tangles have been recognized as two prominent pathological markers for AD [1] , [2] , [3] , [4] , [5] . One emerging consensus is that Aβ oligomers may be the initial trigger for a cascade of responses leading to eventual neurodegeneration [2] , [3] , [6] , [7] . However, clinical trials using γ-secretase inhibitors to reduce Aβ production unexpectedly worsened the symptoms in AD patients [8] , [9] , [10] , prompting a search for new drugs to treat the disorder. γ-aminobutyric acid (GABA) is the major inhibitory neurotransmitter in the adult brain, activating both GABA A and GABA B receptors. GABA A receptors (GABA A -Rs) localize at both synaptic and extrasynaptic sites, mediating phasic and tonic inhibition, respectively [11] , [12] , [13] , [14] . Altered GABAergic function has been reported in AD patients as well as transgenic AD mouse models. For example, recent immunohistochemistry studies revealed a significant reduction in GABAergic nerve terminals in human AD brains [15] . In the hAPP J20 mouse model for AD, a sodium channel Nav1.1 was found depleted in parvalbumin interneurons, leading to reduced activity-dependent GABAergic input and increased network hyperactivity [16] . However, how GABAergic alterations lead to cognitive deficits in AD brains is largely understudied. We investigated GABA function in the dentate gyrus (DG), the gateway for information input to the hippocampus, a critical brain region involved in learning and memory. We discovered unusually high GABA content in the reactive astrocytes of DG in a transgenic mouse model for AD (5xFAD [17] ) as well as in brain samples from human AD patients. Reactive astrocytes are hypertrophic glial cells with elevated level of glial fibrillary acidic protein (GFAP) that are typically activated by injury or diseases [18] . The high GABA content in reactive astrocytes was released by astrocyte-specific GABA transporter GAT3/4 (human GAT3/mouse GAT4) and led to enhanced tonic inhibition in dentate granule cells. Interestingly, the α5-subunit-containing GABA A -Rs (α5-GABA A -Rs) were upregulated in the dentate granule cells of 5xFAD mice, further increasing tonic inhibition therein. As expected, the 5xFAD mice showed impairment in long-term potentiation (LTP) and memory deficit; reducing tonic inhibition in 5xFAD animals rescued the LTP impairment and memory deficit. Our results suggest that increased tonic GABA inhibition in the DG may contribute to functional deficit in AD brains, and astrocytic GABA transporters may serve as a novel drug target for therapeutic intervention. Increased GABA content in dentate astrocytes of 5xFAD mice To investigate the functional role of GABA in AD, we employed a rapid onset mouse model for AD, the 5xFAD mice (APPSwFlLon, PSEN1*M146L*L286V) [17] . Previous studies demonstrated that 5xFAD mice manifest symptoms similar to those of human AD patients, such as Aβ plaques, decreased synaptic proteins, increased reactive astrocytes and memory deficit in the Y-maze [17] . Examination of the Aβ1-42 level in the hippocampus of 5xFAD animals revealed substantially more Aβ1-42 deposits ( Fig. 1a , left panels, red) as well as many more GFAP-labelled reactive astrocytes ( Fig. 1a , green) in the DG than in the CA1 region. Quantitatively, the total areas covered by Aβ1-42 or GFAP immunostaining were significantly larger in the DG than in the CA1 region of 5xFAD brain ( Fig. 1b ). Thus, DG in 5xFAD brain is loaded with heavy Aβ1-42 deposits and massive numbers of reactive astrocytes. This led us to investigate potential GABA functional deficits in the DG of 5xFAD brain. 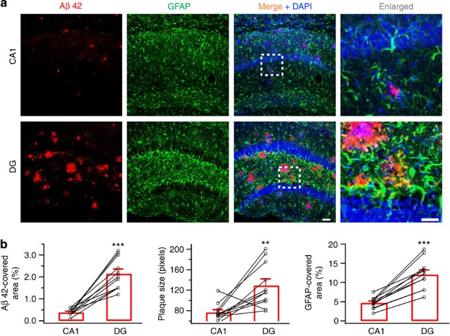Figure 1: DG has more Aβ deposit and reactive astrocytes than the CA1 region in the 5xFAD mice. (a) Representative images showing more Aβ immunostaining (red) and reactive astrocytes (green) in the DG than in the CA1 region of 5xFAD mice. Blue is 4′,6-diamidino-2-phenylindole staining for the cell nucleus. (b) Quantified data showing increased Aβ-covered area, Aβ plaque size and GFAP-covered area in the DG compared with the CA1 region in 5xFAD mice. Bar values are shown as mean±s.e.m.,n=11. Scale bar=50 μm (20 μm in enlarged images). **P<0.01; ***P<0.001; paired Student’st-test. Figure 1: DG has more Aβ deposit and reactive astrocytes than the CA1 region in the 5xFAD mice. ( a ) Representative images showing more Aβ immunostaining (red) and reactive astrocytes (green) in the DG than in the CA1 region of 5xFAD mice. Blue is 4′,6-diamidino-2-phenylindole staining for the cell nucleus. ( b ) Quantified data showing increased Aβ-covered area, Aβ plaque size and GFAP-covered area in the DG compared with the CA1 region in 5xFAD mice. Bar values are shown as mean±s.e.m., n =11. Scale bar=50 μm (20 μm in enlarged images). ** P <0.01; *** P <0.001; paired Student’s t -test. Full size image The imbalance of glutamate excitation and GABA inhibition has been associated with many neurological disorders including AD [16] , [19] . We performed immunostaining of glutamate and GABA in the DG and found no significant difference between wild type (WT) and 5xFAD brains in 3- to 4-month-old animals ( Fig. 2a ). Likewise at this young adult stage, no significant Aβ plaques were detected when examined with thioflavin-s staining in the 5xFAD animals ( Fig. 2a , merged image). However, 6- to 8-month-old 5xFAD animals displayed a remarkable increase in both GABA and glutamate levels in the GFAP-labelled hypertrophic reactive astrocytes in the DG ( Fig. 2b ). These reactive astrocytes were intermingled with Aβ plaques labelled by thioflavin-s staining ( Fig. 2b , merged image, blue). Since GABA is typically converted from glutamate by glutamic acid decarboxylase (GAD), we examined GAD67, a major GABA synthesis enzyme in the nervous system, and found that it increased significantly in the reactive astrocytes in the DG of 5xFAD mice ( Fig. 2c ). Quantitative analysis showed a clear increase in GABA, glutamate and GAD67 in dentate astrocytes in 5xFAD as compared with WT animals ( Fig. 2d ). 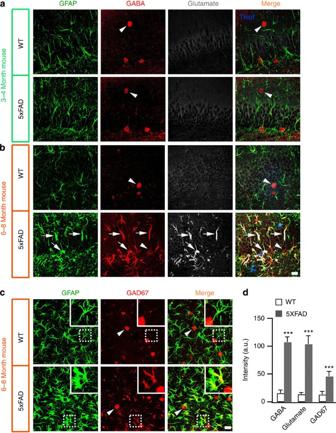Figure 2: High GABA content in the reactive astrocytes of DG in 5xFAD mice. (a) In young adult animals (3–4 months old), both WT and 5xFAD astrocytes (GFAP, green) showed little GABA (red) or glutamate (white) immunoreactivity. Note that GABA immunostaining labelled GABAergic neuronal soma clearly (arrowhead). There were no Aβ plaques detected with thioflavin-s staining (merged image, blue) at this early stage. (b) By 6–8 months of age, WT animals (top row) still showed low level of GABA (red) and glutamate (white) staining in GFAP-labelled astrocytes (green). However, in 5xFAD animals (bottom row), astrocytes (GFAP, green) in the DG showed hypertrophic morphology with strong GABA and glutamate immunostaining. Arrow points to astrocyte; arrowhead points to GABAergic neuron. In merged image, Aβ plaques were labelled by thioflavin-s staining (blue). (c) Higher expression of GAD67 (red) in the DG astrocytes (green) in 5xFAD animals. Scale bar=20 μm. (d) Quantified data showing significant increase in GABA, glutamate and GAD67 in the reactive astrocytes of 5xFAD animals. For GABA and glutamate staining,n=6 WT mice and 7 AD mice. For GAD67 staining,n=4 mice in both groups. Data are presented as mean±s.e.m., ***P<0.001; Student’st-test. Figure 2: High GABA content in the reactive astrocytes of DG in 5xFAD mice. ( a ) In young adult animals (3–4 months old), both WT and 5xFAD astrocytes (GFAP, green) showed little GABA (red) or glutamate (white) immunoreactivity. Note that GABA immunostaining labelled GABAergic neuronal soma clearly (arrowhead). There were no Aβ plaques detected with thioflavin-s staining (merged image, blue) at this early stage. ( b ) By 6–8 months of age, WT animals (top row) still showed low level of GABA (red) and glutamate (white) staining in GFAP-labelled astrocytes (green). However, in 5xFAD animals (bottom row), astrocytes (GFAP, green) in the DG showed hypertrophic morphology with strong GABA and glutamate immunostaining. Arrow points to astrocyte; arrowhead points to GABAergic neuron. In merged image, Aβ plaques were labelled by thioflavin-s staining (blue). ( c ) Higher expression of GAD67 (red) in the DG astrocytes (green) in 5xFAD animals. Scale bar=20 μm. ( d ) Quantified data showing significant increase in GABA, glutamate and GAD67 in the reactive astrocytes of 5xFAD animals. For GABA and glutamate staining, n =6 WT mice and 7 AD mice. For GAD67 staining, n =4 mice in both groups. Data are presented as mean±s.e.m., *** P <0.001; Student’s t -test. Full size image High GABA concentration in 5xFAD hippocampal tissue To independently verify that GABA content is indeed increased in the hippocampus of 5xFAD brain, we developed a novel method to assay GABA concentration in brain homogenate. We first transfected HEK293T cells with GABA A -R α2β3γ2 subunits for detecting GABA responses [11] , [12] . The hippocampal region was dissected out from WT or 5xFAD brain and made into homogenate by repeated freeze and thaw and sonication. The homogenate was then diluted 100-fold and puffed on HEK cells expressing GABA A -Rs (24–48 h after transfection) to assay GABA responses. To validate the method, which we named brain homogenate puff (BHP) assay, we carried out a series of control experiments. First, we puffed brain homogenate on non-transfected HEK cells and found no responses ( Supplementary Fig. 1a ). Second, we puffed bath solution on GABA A -R-expressing HEK cells and also observed no responses ( Supplementary Fig. 1b ). Third, we demonstrated that puffing GABA on GABA A -R-expressing HEK cells evoked large inward currents, which were blocked by GABA A -R antagonist bicuculline (BIC, 50 μM; Supplementary Fig. 1c ). Similarly, puffing hippocampal homogenate on GABA A -R-expressing HEK cells also evoked a significant current, which was blocked by BIC as well ( Supplementary Fig. 1d ). Fourth, in order to compare WT and 5xFAD brain homogenate side by side, we filled a bundle of triple identical micropipettes with WT homogenate, GABA (10 μM, determined after pilot experiments; in the middle) and 5xFAD homogenate ( Fig. 3a ). When the three micropipettes were filled with the same concentration of GABA, they evoked the same size of GABA responses ( Fig. 3b,c ). Similarly, when they were filled with the same brain homogenate, either from WT or 5xFAD hippocampal tissue, they evoked the same size of GABA responses ( Supplementary Fig. 1e–h ). Alternatively, when the three micropipettes were filled with different concentrations of GABA (1, 3 and 10 μM), they evoked different sizes of GABA responses ( Fig. 3d,f ). After these rigorous control experiments, we tested GABA responses in the same HEK cells expressing GABA A -Rs by puffing WT and 5xFAD hippocampal homogenate, together with 10 μM GABA. We found that the 5xFAD hippocampal homogenate consistently evoked larger GABA responses than the WT counterpart ( Fig. 3g–i ). Quantitatively, the GABA current evoked by 5xFAD hippocampal homogenate was about twice as large as that evoked by WT hippocampal homogenate ( Fig. 3j ; WT, 363.7±99.2 pA; 5xFAD, 637.1±84.5 pA; n =3 sets, total 24 cells; P <0.03; paired Student’s t -test). After normalization, WT hippocampal homogenate-evoked GABA current was 39.1±8.7%, whereas the 5xFAD hippocampal homogenate-evoked GABA current was 72.7±2.1% of that evoked by 10 μM GABA ( Fig. 3k ). In addition to electrophysiology assay, we further performed GABA ELISA assay to quantitatively measure the GABA concentration in hippocampal tissue from WT or 5xFAD mice. Interestingly, young animals (3–4 months old) did not show any difference in GABA content (WT, 0.41±0.01 μg mg −1 , n =6; 5xFAD, 0.42±0.02 μg mg −1 , n =5; P >0.6) but old 5xFAD mice (7–8 months old) showed significantly increased GABA content in hippocampal homogenate ( Fig. 3l ; WT, 0.41±0.03 μg mg −1 , n =5; 5xFAD, 0.55±0.04 μg mg −1 , n =4; P <0.02). Therefore, the hippocampal tissue in 5xFAD mice has higher GABA content than that in WT mice, likely because of the accumulation of GABA in the reactive astrocytes in 5xFAD brains. 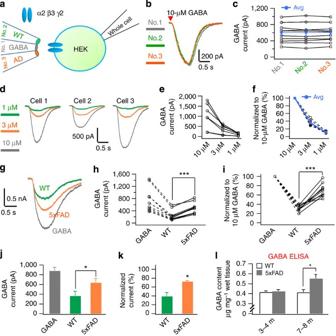Figure 3: Brain homogenate assay detected higher GABA concentration in the hippocampal tissue of 5xFAD mice. (a) Schematic diagram illustrating the experimental arrangement of BHP assay. (b,c) Triple micropipettes filled with the same concentration of GABA (10 μM) evoked the same size of GABA responses in a set of HEK cells expressing different levels of GABAA-Rs. (d–f) Triple micropipettes filled with different concentrations of GABA (1, 3 and 10 μM) evoked different sizes of GABA responses in HEK cells. (g–i) A typical set of experiments showing responses evoked by WT or AD hippocampal homogenate and GABA (10 μM) in HEK cells expressing GABAA-Rs. Note that AD hippocampal homogenate always evoked larger GABA responses in the same cell than that from WT littermate. (j,k) Quantitative data showing increased GABA current amplitude evoked by hippocampal homogenate from 5xFAD mice compared with that from WT mice (n=3 sets, total 24 cells). (l) GABA ELISA assay showing that GABA concentration in the hippocampal tissue increased significantly in old 5xFAD mice (7–8 months,n=5 mice for WT;n=4 mice for 5xFAD) but not in young animals (3–4 months,n=6 mice for WT;n=5 mice for 5xFAD). Note that GABA concentration did not change in WT animals. Data are presented as mean±s.e.m., *P<0.05; **P<0.01; ***P<0.001; Student’st-test. Figure 3: Brain homogenate assay detected higher GABA concentration in the hippocampal tissue of 5xFAD mice. ( a ) Schematic diagram illustrating the experimental arrangement of BHP assay. ( b , c ) Triple micropipettes filled with the same concentration of GABA (10 μM) evoked the same size of GABA responses in a set of HEK cells expressing different levels of GABA A -Rs. ( d – f ) Triple micropipettes filled with different concentrations of GABA (1, 3 and 10 μM) evoked different sizes of GABA responses in HEK cells. ( g – i ) A typical set of experiments showing responses evoked by WT or AD hippocampal homogenate and GABA (10 μM) in HEK cells expressing GABA A -Rs. Note that AD hippocampal homogenate always evoked larger GABA responses in the same cell than that from WT littermate. ( j , k ) Quantitative data showing increased GABA current amplitude evoked by hippocampal homogenate from 5xFAD mice compared with that from WT mice ( n =3 sets, total 24 cells). ( l ) GABA ELISA assay showing that GABA concentration in the hippocampal tissue increased significantly in old 5xFAD mice (7–8 months, n =5 mice for WT; n =4 mice for 5xFAD) but not in young animals (3–4 months, n =6 mice for WT; n =5 mice for 5xFAD). Note that GABA concentration did not change in WT animals. Data are presented as mean±s.e.m., * P <0.05; ** P <0.01; *** P <0.001; Student’s t -test. Full size image High GABA content in dentate astrocytes of human AD brains Reactive astrocytes have been widely reported in neurodegenerative disorders including AD [20] , [21] . However, such high levels of GABA found in the reactive astrocytes of 5xFAD mouse brain are unexpected. To ensure that this is not an artifact only found in transgenic AD animal models, we examined human hippocampal tissue from post-mortem AD patients (Emory Brain Bank, sample information in Supplementary Table 1 ). Consistent with the finding in 5xFAD mice, we found a substantial accumulation of GABA in GFAP-labelled astrocytes in the DG (molecular layer) in AD patients but not healthy controls ( Fig. 4a , quantified in Fig. 4c , P <0.001). Similarly, the level of GAD67 also significantly increased in the DG-reactive astrocytes of AD patients ( Fig. 4b , quantified in Fig. 4c , P <0.001). These results suggest that the high GABA level in the reactive astrocytes of AD brains may serve as a novel biomarker for AD. 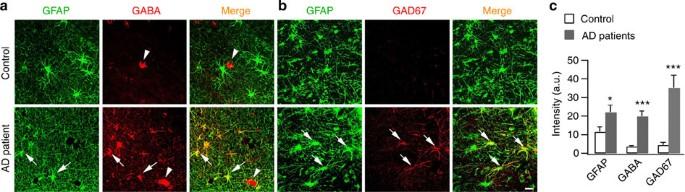Figure 4: Human hippocampal tissue from AD patients showed higher GABA content in reactive astrocytes. (a) GABA immunostaining (red) in the molecular layer of DG in human hippocampal tissue. Control human astrocytes (GFAP, green) showed little GABA staining (top row), whereas astrocytes from AD patients showed significant amount of GABA staining (arrow). Arrowhead points to GABAergic neuron.n=9 for both control and AD groups. (b) Representative images showing increased GAD67 immunosignal (red) in human hippocampal astrocytes (green) from AD patients compared with controls.n=6 for both control and AD groups. Scale bar=20 μm. (c) Quantified data showing significant increase in GFAP, GABA and GAD67 in dentate astrocytes from human AD patients (data are shown as mean±s.e.m.). *P<0.05; ***P<0.001; Student’st-test. Figure 4: Human hippocampal tissue from AD patients showed higher GABA content in reactive astrocytes. ( a ) GABA immunostaining (red) in the molecular layer of DG in human hippocampal tissue. Control human astrocytes (GFAP, green) showed little GABA staining (top row), whereas astrocytes from AD patients showed significant amount of GABA staining (arrow). Arrowhead points to GABAergic neuron. n =9 for both control and AD groups. ( b ) Representative images showing increased GAD67 immunosignal (red) in human hippocampal astrocytes (green) from AD patients compared with controls. n =6 for both control and AD groups. Scale bar=20 μm. ( c ) Quantified data showing significant increase in GFAP, GABA and GAD67 in dentate astrocytes from human AD patients (data are shown as mean±s.e.m.). * P <0.05; *** P <0.001; Student’s t -test. Full size image Increased astrocytic GABA transporter in AD brains GABA is mainly synthesized from glutamate by GAD. Alternatively, GABA may also be uptaken through GABA transporters. Astrocytes have unique GABA transporters that are distinctly different from neuronal GABA transporters (GAT1) [22] . GAT4 is the major isoform of astroglial GABA transporter in mouse, while its orthologue in human and rat is GAT3, and GAT3/4 is often used when more than one species is studied together. We found a significant increase in GAT3/4 in the reactive astrocytes of DG in 5xFAD mice ( Fig. 5a ; WT, 15.7±3.6 a.u., n =6; AD, 66±14 a.u., n =6; P <0.01, Student’s t -test). Such elevated levels of GAT3/4 were further confirmed in the reactive astrocytes of DG in human AD brains ( Fig. 5b ; control, 16.0±1.5 a.u., n =6; AD patients, 44.2±1.7 a.u., n =6; P <0.001). Thus, the astrocytic GABA transporter GAT3/4 is significantly increased in both human and mouse AD brains. 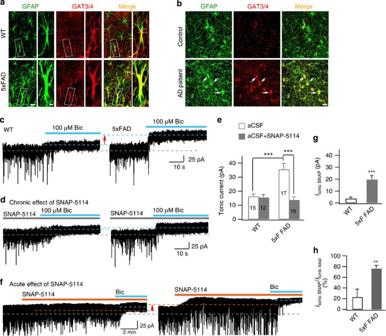Figure 5: Increase in GAT3/4 in AD-reactive astrocytes and contribution towards enhanced tonic GABA current in dentate granule cells. (a) Significant increase in GAT3/4 immunoreactivity (red) in the dentate astrocytes (GFAP, green) in 5xFAD animals (bottom row), compared with controls (top row).n=6 mice for WT or AD group. Scale bar=20 μm (5 μm in enlarged image). (b) Human dentate astrocytes (GFAP, green) in AD patients (bottom row) also showed remarkable increase in GAT3/4 staining (red, arrow).n=6 for both control and AD groups. Scale bar=20 μm. (c) Dentate granule cells in 5xFAD animals (right panel) showed enhanced tonic current, revealed by GABAA-R antagonist BIC, compared with controls (left panel). (d) Chronic blockade of GAT3/4 with specific inhibitor SNAP-5114 (50 μM, 2 h) significantly diminished the tonic current in dentate granule cells in 5xFAD animals (right panel), compared with that in WT mice (left panel). Synaptic currents were truncated for better view of the small tonic current. (e) Quantified data ofc,d(analysis of variance (ANOVA) with Tukeypost hoctests) and cell number is shown in histograms. (f) Acute application of SNAP-5114 also blocked the majority of the tonic current in dentate granule cells in 5xFAD animals but showed little effect in WT dentate granule cells. (g,h) Quantified data inf, showing a major contribution of GAT3/4 towards the tonic current in 5xFAD dentate granule cells (Student’st-test).n=12 for WT and 13 for 5xFAD group. Data are presented as mean±s.e.m., **P<0.01; ***P<0.001. Figure 5: Increase in GAT3/4 in AD-reactive astrocytes and contribution towards enhanced tonic GABA current in dentate granule cells. ( a ) Significant increase in GAT3/4 immunoreactivity (red) in the dentate astrocytes (GFAP, green) in 5xFAD animals (bottom row), compared with controls (top row). n =6 mice for WT or AD group. Scale bar=20 μm (5 μm in enlarged image). ( b ) Human dentate astrocytes (GFAP, green) in AD patients (bottom row) also showed remarkable increase in GAT3/4 staining (red, arrow). n =6 for both control and AD groups. Scale bar=20 μm. ( c ) Dentate granule cells in 5xFAD animals (right panel) showed enhanced tonic current, revealed by GABA A -R antagonist BIC, compared with controls (left panel). ( d ) Chronic blockade of GAT3/4 with specific inhibitor SNAP-5114 (50 μM, 2 h) significantly diminished the tonic current in dentate granule cells in 5xFAD animals (right panel), compared with that in WT mice (left panel). Synaptic currents were truncated for better view of the small tonic current. ( e ) Quantified data of c , d (analysis of variance (ANOVA) with Tukey post hoc tests) and cell number is shown in histograms. ( f ) Acute application of SNAP-5114 also blocked the majority of the tonic current in dentate granule cells in 5xFAD animals but showed little effect in WT dentate granule cells. ( g , h ) Quantified data in f , showing a major contribution of GAT3/4 towards the tonic current in 5xFAD dentate granule cells (Student’s t -test). n =12 for WT and 13 for 5xFAD group. Data are presented as mean±s.e.m., ** P <0.01; *** P <0.001. Full size image Enhanced tonic inhibition in the DG of 5xFAD mice The high levels of astrocytic GAT3/4 can either uptake GABA into, or transport GABA outside of, astrocytes. Astrocytes have been shown to reverse GABA transporter to release GABA if stimulated by glutamate [23] . Since glutamate excitotoxicity is well documented in the AD mouse models [24] , we tested whether GAT3/4 in the reactive astrocytes of 5xFAD mice is capable of releasing GABA. If GABA is released by reactive astrocytes in the DG, the most sensitive detector will be the extrasynaptic GABA A -Rs in dentate granule cells, which have high affinity for GABA and will result in tonic GABA current when activated by ambient GABA [13] . Therefore, we performed patch clamp recordings in mouse hippocampal slices to record tonic GABA currents ( I Tonic ) in dentate granule cells. In WT mice (6–8 months old), we detected a small tonic GABA current in dentate granule cells ( Fig. 5c , left panel). However, in the dentate granule cells of 5xFAD animals (6–8 months old), the tonic current was significantly larger ( Fig. 5c , right panel). To investigate whether this enhanced tonic GABA current is causally linked to the increased astrocytic GABA transporter, we incubated 5xFAD hippocampal slices with GAT3/4 inhibitor SNAP-5114 (50 μM) for 2 h. Chronically blocking GAT3/4 activity had no effect on WT dentate granule cells ( Fig. 5d , left panel), but significantly diminished the tonic GABA current in 5xFAD dentate granule cells ( Fig. 5d , right panel; quantified in Fig. 5e ; P <0.001). Acute application of SNAP-5114 (50 μM) also reduced tonic GABA current in 5xFAD dentate granule cells ( Fig. 5f , quantified in Fig. 5g,h ), suggesting that astrocytic GABA release may contribute significantly towards tonic inhibition in 5xFAD brains. As a control, we recorded tonic GABA current in the dentate granule cells in young adult animals (3–4 months old) but found no difference between WT and 5xFAD individuals ( Supplementary Fig. 2a,b ; WT, 16.4±1.3 pA, n =16; 5xFAD, 16.5±1.6 pA, n =15; P >0.9), consistent with the very low level of GABA immunostaining in astrocytes of young adult animals ( Fig. 2a ). We further investigated whether neuronal GABA transporter GAT1 might be altered in 5xFAD mice. Application of a GAT1-specific blocker NO-711 (10 μM) revealed large tonic currents in both WT and 5xFAD animals with no significant difference ( Supplementary Fig. 2c,d ; WT, 97±20 pA, n =8; 5xFAD, 112±18 pA, n =7; P >0.4). Importantly, blocking GAT3/4 decreased tonic current, whereas blocking GAT1 enhanced tonic current (compare Fig. 5f with Supplementary Fig. 2c ), indicating that GAT3/4 is releasing, whereas GAT1 is uptaking, GABA. Thus, the high GABA content in the reactive astrocytes of 5xFAD brains can be released through GABA transporter GAT3/4 to enhance tonic inhibition in dentate granule cells. Upregulation of α5-GABA A- Rs in 5xFAD dentate granule cells Tonic GABA currents are typically mediated by extrasynaptic GABA A -Rs, including δ subunit- and α5-subunit-containing GABA A -Rs [12] , [13] . We next investigated which subtype of GABA A -Rs mediated the enhanced tonic GABA current in 5xFAD dentate granule cells. The δ subunit-containing GABA A -Rs are known to be expressed in the dentate granule cells [25] . Therefore, we applied THIP (2 μM), a selective agonist for δ-GABA A -Rs (EC50=6.3 μM (ref. 26 )), to examine the tonic current in dentate granule cells in hippocampal slices. Surprisingly, the THIP-induced tonic currents did not show significant difference between WT and 5xFAD dentate granule cells ( Supplementary Fig. 2e,f ; WT, 65.2±6.6 pA, n =8; 5xFAD, 60.7±10.4 pA, n =8; P >0.7). Besides δ-GABA A -Rs, α5-GABA A -Rs were also reported to partially mediate the tonic current in dentate granule cells [14] . We therefore employed α5-specific inverse agonist L-655,708 to examine the contribution from the α5-GABA A -Rs. In WT animals, application of L-655,708 (100 nM) in the presence of 5 μM GABA partially reduced the tonic current in dentate granule cells ( Fig. 6a , left), whereas in 5xFAD mice, L-655,708 blocked the majority of the tonic current activated by 5 μM GABA ( Fig. 6a , right), suggesting a significant contribution of the α5-GABA A -Rs towards tonic inhibition in 5xFAD mice. Quantitatively, the tonic current blocked by L-655,708 in 5xFAD dentate granule cells was more than double of that in WT dentate granule cells ( Fig. 6b ; WT, 35.4±6.3 pA, n =12; 5xFAD, 98.7±12.9 pA, n =9; P <0.001). Since α5-GABA A -Rs are known to be expressed in CA1 pyramidal neurons, we further recorded the tonic current in CA1 region and found similar tonic currents between WT and 5xFAD animals ( Fig. 6c ; WT, 31.2±4.7 pA, n =11; 5xFAD, 36.1±6.7 pA, n =9; P >0.5), and the proportion of tonic current blocked by L-655,708 was also similar in CA1 neurons between WT and 5xFAD animals ( Fig. 6d ). In contrast, the proportion of L-655,708-sensitive tonic current significantly increased in 5xFAD dentate granule cells ( Fig. 6d , P <0.001). These results suggest that the α5-GABA A -Rs are upregulated in the DG of 5xFAD mice. 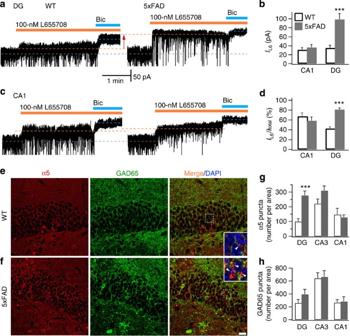Figure 6: Upregulation of α5-GABAAreceptors in the dentate granule cells of 5xFAD animals. (a) Dentate granule cells in WT animals (left) showed a small component of tonic current that was sensitive to the inverse agonist L-655,708 (100 nM) specific for α5-GABAA-Rs, but L-655,708 blocked the majority of tonic current in the dentate granule cells of 5xFAD animals (right). GABA (5 μM) was included in the bath solution to increase the tonic current. (c) CA1 pyramidal neurons showed similar L-655,708-sensitive tonic currents between WT and 5xFAD animals. (b,d) Quantified data showing increased tonic current mediated by the α5-GABAA-Rs in dentate granule cells of 5xFAD animals. (e,f) Double immunostaining of the α5-subunit (red) and GAD65 (green) in the DG revealed a significant increase in α5 puncta in the dentate granule cells of 5xFAD mice. Inset showing that the majority of α5 puncta were extrasynaptic, not colocalizing with presynaptic GAD65 puncta. Scale bar=20 μm. (g,h) Quantified data showing increased α5 puncta number, but not GAD65, in the DG of 5xFAD mice (n=6 mice for WT and 9 mice for 5xFAD group). No differences were found in CA1 or CA3 regions between WT and 5xFAD mice. Data are presented as mean±s.e.m., ***P<0.001, Student’st-test. Figure 6: Upregulation of α5-GABA A receptors in the dentate granule cells of 5xFAD animals. ( a ) Dentate granule cells in WT animals (left) showed a small component of tonic current that was sensitive to the inverse agonist L-655,708 (100 nM) specific for α5-GABA A -Rs, but L-655,708 blocked the majority of tonic current in the dentate granule cells of 5xFAD animals (right). GABA (5 μM) was included in the bath solution to increase the tonic current. ( c ) CA1 pyramidal neurons showed similar L-655,708-sensitive tonic currents between WT and 5xFAD animals. ( b , d ) Quantified data showing increased tonic current mediated by the α5-GABA A -Rs in dentate granule cells of 5xFAD animals. ( e , f ) Double immunostaining of the α5-subunit (red) and GAD65 (green) in the DG revealed a significant increase in α5 puncta in the dentate granule cells of 5xFAD mice. Inset showing that the majority of α5 puncta were extrasynaptic, not colocalizing with presynaptic GAD65 puncta. Scale bar=20 μm. ( g , h ) Quantified data showing increased α5 puncta number, but not GAD65, in the DG of 5xFAD mice ( n =6 mice for WT and 9 mice for 5xFAD group). No differences were found in CA1 or CA3 regions between WT and 5xFAD mice. Data are presented as mean±s.e.m., *** P <0.001, Student’s t -test. Full size image To corroborate the electrophysiology data, we performed immunostaining and detected α5-immunopositive signal in the dentate granule layer ( Fig. 6e ), as reported before [27] . Interestingly, the α5 receptors were significantly increased in 5xFAD dentate granule cells ( Fig. 6f,g ; P <0.001), consistent with the enhanced tonic current mediated by α5-GABA A -Rs. Note that consistent with their typical extrasynaptic localization, the majority of α5 puncta were not colocalized with presynaptic GAD65 puncta ( Fig. 6e,f , inset). GAD67 is the major GABA synthesis enzyme mainly localized in cell bodies, while GAD65 is localized at GABAergic nerve terminals and often used as a presynaptic marker. While the α5 receptors significantly increased in the DG of 5xFAD animals, the GAD65 puncta number did not change in the hippocampus ( Fig. 6h ). Therefore, the α5-GABA A -Rs are upregulated in 5xFAD dentate granule cells and contribute to the enhanced tonic inhibition in the DG. Reducing tonic inhibition rescues the impairment of LTP To investigate the functional consequence of enhanced tonic inhibition in the 5xFAD brain, we examined the LTP in the DG by performing hippocampal slice recordings. WT animals (6–8 months old) showed normal LTP in the DG after high-frequency stimulation (HFS; 100 Hz for 1 s, repeated three times with 20 s interval); however, the same age 5xFAD animals showed significantly decreased LTP ( Fig. 7a , quantified in Fig. 7b ; WT, green; 5xFAD, grey; P <0.01). Interestingly, suppression of tonic inhibition, either with SNAP-5114 (50 μM, blue) to block astrocytic GABA release or with L-655,708 (100 nM, orange) to block α5-GABA A -Rs, rescued the LTP impairment in the 5xFAD dentate granule cells ( Fig. 7a,b , P <0.05). The LTP in the DG of WT animals was not affected by the drug treatment ( Fig. 7b ). Therefore, the enhanced tonic inhibition in the DG of 5xFAD mice may play a critical role in the suppression of LTP. 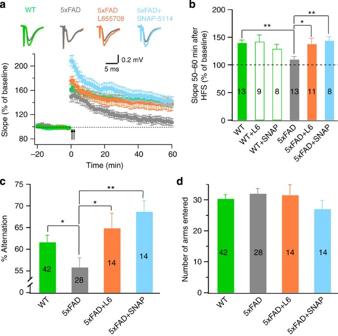Figure 7: Blockade of tonic inhibition rescued deficits in LTP and working memory in 5xFAD mice. (a) Hippocampal slice recordings revealed LTP impairment in the DG of 5xFAD mice (grey), compared with the control animals (green). Blocking tonic inhibition by L-655,708 (100 nM, orange) or SNAP-5114 (50 μM, blue) rescued the impairment of LTP. (b) Quantified potentiation within 50–60 min after high-frequency stimulation in various conditions. Two-way ANOVA revealed a significant change among genotype and drug treatments (F (2, 56)=3.7,P<0.04), numbers in histograms indicate number of slices. (c) Y-maze test showed significant impairment of spontaneous alternation behaviour in 5xFAD mice (grey) compared with WT animals (green). Chronic block of tonic inhibition by repeated injection of L-655,708 or SNAP-5114 for 1 week rescued the behavioural deficit. (d) The total number of arm entries were not different among WT, 5xFAD, 5xFAD+L-655,708 and 5xFAD+SNAP-5114 groups. Numbers in histograms (c,d) indicate number of mice. Data are presented as mean±s.e.m., *P<0.05; **P<0.01. Figure 7: Blockade of tonic inhibition rescued deficits in LTP and working memory in 5xFAD mice. ( a ) Hippocampal slice recordings revealed LTP impairment in the DG of 5xFAD mice (grey), compared with the control animals (green). Blocking tonic inhibition by L-655,708 (100 nM, orange) or SNAP-5114 (50 μM, blue) rescued the impairment of LTP. ( b ) Quantified potentiation within 50–60 min after high-frequency stimulation in various conditions. Two-way ANOVA revealed a significant change among genotype and drug treatments (F (2, 56)=3.7, P <0.04), numbers in histograms indicate number of slices. ( c ) Y-maze test showed significant impairment of spontaneous alternation behaviour in 5xFAD mice (grey) compared with WT animals (green). Chronic block of tonic inhibition by repeated injection of L-655,708 or SNAP-5114 for 1 week rescued the behavioural deficit. ( d ) The total number of arm entries were not different among WT, 5xFAD, 5xFAD+L-655,708 and 5xFAD+SNAP-5114 groups. Numbers in histograms ( c , d ) indicate number of mice. Data are presented as mean±s.e.m., * P <0.05; ** P <0.01. Full size image We further investigated the effect of tonic current on cell excitability in WT and 5xFAD dentate granule cells ( Supplementary Fig. 3 ). It is known that dentate granule cells do not fire spontaneous action potentials (APs) because of hyperpolarized resting membrane potentials (typically −80 mV, Supplementary Fig. 3a–c ). The intrinsic membrane conductance was found to be similar between WT and 5xFAD dentate granule cells ( Supplementary Fig. 3d–e ). We then injected currents (~70 pA) to make granule cells firing APs, similar to previously published work [28] , [29] . When 5 μM GABA was applied in the bath solution to activate tonic GABA currents, we found that WT granule cells showed little change in AP firing, but 5xFAD granule cells showed a significant decrease in AP firing ( Supplementary Fig. 3f,g , quantified in h; P <0.001), consistent with the increased tonic current in 5xFAD granule cells ( Fig. 6a ). Importantly, blocking tonic current with the α5 GABA A -R inverse agonist L-655,708 rescued the AP firing in 5xFAD granule cells ( Supplementary Fig. 3g,h ; P <0.001), confirming an increased tonic inhibition in the DG of 5xFAD mice. In addition, blocking all GABA A -R-mediated inhibition with 100 μM picrotoxin increased AP firing in both WT and 5xFAD granule cells ( Supplementary Fig. 3f–h ), as expected. These results suggest that the enhanced tonic inhibition in the DG of 5xFAD mice plays a critical role in regulating neuronal activity. Reducing tonic inhibition alleviates memory deficit We further conducted behavioural analysis to test the effect of enhanced tonic inhibition on the cognitive function of 5xFAD animals. It has been reported that 5xFAD mice show a significant memory deficit in the spontaneous alternation test in Y-maze [17] . We first confirmed that our 5xFAD mice indeed showed such memory deficit when placed in a Y-maze to test their sequential entries in each arm ( Fig. 7c , P <0.05). Interestingly, intraperitoneal administration of SNAP-5114 (50 μmol kg −1 , i.p., once per day for 1 week; blue) or L-655,708 (1 mg kg −1 , i.p., once per day for 1 week; orange) rescued the memory deficit in 5xFAD animals ( Fig. 7c , P <0.05). The total number of arm entry did not differ among WT, 5xFAD and 5xFAD plus drug treatment groups ( Fig. 7d ). Therefore, we conclude that the enhanced tonic inhibition in the DG of 5xFAD mice contributes to the impairment of memory. Our studies discovered unusual GABA accumulation in the reactive astrocytes in the DG of both mouse and human AD brains, leading to enhanced tonic GABA inhibition. Functional and behavioural analyses demonstrated that such increased tonic inhibition suppresses LTP and results in memory deficit in 5xFAD animals. On the basis of these results, we propose a working model ( Fig. 8 ) that in the DG of AD brains, excitotoxic/inflammatory stimulation, possibly originated from Aβ deposit, will stimulate reactive astrocytes to accumulate glutamate and convert it into GABA. The high level of GABA in reactive astrocytes will be released through GAT3/4 to increase ambient GABA concentration in the DG of AD brain. In the meanwhile, the α5-GABA A -Rs in AD dentate granule cells are upregulated to further enhance tonic inhibition. This increased tonic inhibition in the AD brain may initially be part of a compensatory mechanism to antagonize glutamate excitotoxicity. However, chronic increase of tonic inhibition in the DG of AD brain will suppress LTP and result in learning and memory deficits. Our studies suggest that reducing tonic inhibition in the DG of AD brains may lead to a potential new therapy for AD. 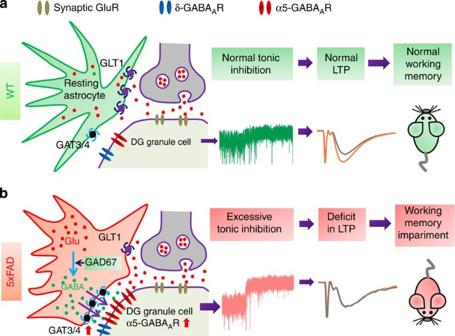Figure 8: Working model. (a) WT animals have normal level of GABA, glutamate and GAT3/4 in astrocytes, and normal level of δ- and α5-GABAA-Rs in dentate granule cells. The tonic inhibition is small. There is significant LTP in the DG, and animals have normal cognitive functions. (b) 5xFAD animals show abnormally high level of glutamate, GABA and GAT3/4 in the reactive astrocytes, and upregulated α5-GABAA-Rs in dentate granule cells. The tonic inhibition is significantly enhanced, and LTP in the DG is suppressed. Animals display learning and memory deficits. Figure 8: Working model. ( a ) WT animals have normal level of GABA, glutamate and GAT3/4 in astrocytes, and normal level of δ- and α5-GABA A -Rs in dentate granule cells. The tonic inhibition is small. There is significant LTP in the DG, and animals have normal cognitive functions. ( b ) 5xFAD animals show abnormally high level of glutamate, GABA and GAT3/4 in the reactive astrocytes, and upregulated α5-GABA A -Rs in dentate granule cells. The tonic inhibition is significantly enhanced, and LTP in the DG is suppressed. Animals display learning and memory deficits. Full size image Astrocytes play a variety of functions in the brain including regulation of neuronal connectivity and activity, participation in the brain–blood barrier and maintenance of energy and ionic balance [30] , [31] . Astrocytes regulate neuronal synapse formation during brain development [32] and also form tripartite synapses with neurons [33] , uptake glutamate released by nerve terminals and convert into glutamine to shuttle back to neurons [34] . Compared with the well-studied astrocytic glutamate–glutamine cycle, astrocytic GABA and GABA transporters are understudied, particularly in neurological disorders. Astrocytes are reported to be immunoreactive for GABA and can also release GABA [35] , [36] , [37] , [38] , [39] . Our present study suggests that astrocytes may have very low level of GABA in the adult brain under physiological conditions, compared with the high level of GABA immunostaining in GABAergic neurons. However, under pathological conditions such as AD, reactive astrocytes start to accumulate a significant amount of GABA. Consistent with our study, GABA immunostaining also increases significantly in reactive astrocytes after ischaemic insult [40] . Notably, we observed no significant change in astrocytic GABA content in young adult 5xFAD mice, which also lack Aβ plaques. By the age of 6–8 months, Aβ plaques were spreading throughout the DG of 5xFAD mice and astrocytic GABA content increased dramatically, suggesting a progressive accumulation of astrocytic GABA that might correlate with Aβ pathology. Astrocytes may uptake GABA through astrocyte-specific GABA transporter GAT3/4 (ref. 41 ). Alternatively, they may convert glutamate into GABA through GAD67. Astrocytic glutamate is normally converted into glutamine by glutamine synthetase. However, it is widely reported that glutamine synthetase is significantly reduced under pathological conditions [31] . Our study discovered that GAD67 can be upregulated in AD-reactive astrocytes; a possible compensation for the reduction of glutamine synthetase in order to process glutamate accumulated in astrocytes. In agreement with our study, an increased GABA synthesis in astrocytes has been reported in a different transgenic mouse model for AD [42] . Therefore, high levels of astrocytic GABA content may be a novel biomarker for brain pathology including AD. The GABA accumulation in the reactive astrocytes of 5xFAD mice seems to have reached a significant level that can be detected by GABA ELISA or a newly developed BHP assay. Both assays demonstrated that the 5xFAD hippocampal tissue has higher GABA content than WT hippocampal tissue. It should be noted that GABA concentration in brain homogenate is the summation of total GABA in both astrocytes and neurons. Under normal conditions, GABAergic neurons may contain the majority of GABA in brain tissue. However, under pathological conditions such as AD, high GABA content in reactive astrocytes may account for a substantial proportion. Nevertheless, if GABAergic neurons degenerate significantly such as at the late stages of AD, the total GABA content in the brain homogenate might reduce. Therefore, the net GABA level in brain tissue may vary under different pathological conditions, or even change at different stages of the same disease. In contrast, GABA content in reactive astrocytes may be a better pathological marker than the total GABA concentration in the brain tissue. The high GABA content in AD-reactive astrocytes has to be released to accommodate newly converted GABA from glutamate. One study reports that cerebellar glial cells may release GABA through an anion channel Bestrophin 1 (ref. 36 ). Alternatively, GABA transporter in astrocytes may reverse its direction to release GABA under stimulation of glutamate [37] . Indeed, GABA transporter has been reported to reverse its transport direction under both physiological and pathological conditions [43] . In the adult hippocampus, GABA uptake is mainly mediated by GAT1, the major GABA transporter in neurons [44] . In accordance, we demonstrated that blocking GAT1 with NO-711 induced a large tonic current in WT animals, indicating an increase in ambient GABA because of the blockage of GABA uptake by GAT1. In contrast, blocking astrocytic GAT3/4 with SNAP-5114 induced no significant change in tonic current in WT animals. In 5xFAD animals, however, blocking GAT3/4 reduced rather than increased tonic current, suggesting that GAT3/4 in 5xFAD-reactive astrocytes normally releases GABA to increase ambient GABA concentration. Since the expression level of GAT3/4 is significantly increased in AD-reactive astrocytes, both in 5xFAD animals and human AD patients, we propose that GAT3/4 may serve as a novel drug target for developing a new therapy to treat AD. The GABA A -R α5-subunit is widely expressed in the early-embryonic brain and later restricted to the hippocampus and olfactory bulb in the adult brain [45] . The α5-GABA A -Rs are known to be involved in learning and memory because of their specific localization in the hippocampus [46] , [47] , [48] . GABA inhibition, including tonic inhibition mediated by α5-GABA A -Rs, has been reported to affect the induction and maintenance of LTP [49] , [50] , [51] , [52] . Our studies demonstrate that α5-GABA A -Rs are upregulated in the DG of 5xFAD animals and blocking α5-GABA A -Rs rescues the impairment of LTP and memory deficit. Consistent with our finding, the α5-GABA A -Rs have been found to enhance the tonic inhibition after stroke [53] and are involved in the inflammation-induced memory deficit [54] . Therefore, α5-GABA A -Rs may serve as a common pathological marker for both brain injury and neurological disorders. However, inverse agonists of α5-GABA A -Rs, developed for the purpose of treating human memory deficit, failed clinical trials [55] , possibly because of their potential side effect on other synaptic GABA A -Rs. This may make the astrocytic GABA transporter GAT3/4 a more attractive drug target because GAT3/4 inhibitors are more specific to astrocytes and may have fewer side effects on neurons. The DG is the gateway to the hippocampus, playing an important role in detecting, sorting and encoding information input from the entorhinal cortex. Compared with other hippocampal areas, the DG of 5xFAD animals has higher level of Aβ deposit and more reactive astrocytes. The high level of Aβ deposit in DG suggests that DG is subjected to severe excitotoxic and inflammatory stimulation. The reactive astrocytes are likely a reaction to the Aβ stimulation and may play both a detrimental and neuroprotective role in the AD brain [18] , [56] , [57] . We demonstrate here that reactive astrocytes in the 5xFAD brain have high GABA content, which enhances tonic inhibition in DG. This increased tonic inhibition may be the result of Aβ stimulation in order to offset glutamate excitotoxicity. The upregulation of α5-GABA A -Rs may also be a compensatory mechanism to reduce excitotoxicity in DG. While tonic inhibition may initially exert a neuroprotective role, chronic enhancement of tonic inhibition in DG will eventually impair LTP and cognitive functions in AD brains, possibly through suppressing AP firing. Therefore, while Aβ and other factors may trigger the initial neurodegenerative process, it is important to correct the downstream changes, such as the increased tonic inhibition discovered in this study, to effectively treat AD. Our study may offer a potential explanation as to why simply reducing Aβ production in AD patients may not have worked in clinical trials. One of the reasons might be that the downstream alterations that are already triggered by Aβ deposit cannot be corrected by reducing Aβ production, at least not easily. We propose here that reducing tonic inhibition may offer a novel treatment for AD patients. Experimental animals The 5xFAD transgenic mice were purchased from the Jackson Laboratory (stock number: 006554), carrying mutations on both human APP (Swedish (K670N/M671L), Florida (I716V) and London (V717I)) and human PS1 proteins (M146L and L286V) [17] . This transgenic line was crossed with the C57BL/6 mice for breeding. Both male and female mice at the age of 6–8 months (5xFAD and age-matched WT littermates) were used in the present study. Young adult mice at the age of 3–4 month were also used as control. Mice were housed in a 12-h light–dark cycle and supplied with food and water. Experimental protocols were approved by Pennsylvania State University IACUC, in accordance with the guidelines of the National Institutes of Health for the Care and Use of Laboratory Animals. Human case material Human hippocampal tissues were provided by the Emory University Alzheimer’s Disease Center and Center for Neurodegenerative Disease Brain Bank from nine cases meeting CERAD [58] , NIA-Reagan [59] and National Institute on Aging-Alzheimer’s Association [60] criteria for the neuropathologic diagnosis of AD (see Supplementary Table 1 for case information). Tissue from nine controls with no history of neurological disease and no significant neuropathologic changes was also provided. Immunohistochemistry For mouse brain tissue immunostaining, mice were deeply anaesthetized with 2.5% Avertin and then perfused with saline solution (0.9% NaCl) to wash off blood in the brain, followed by perfusing ice-cold 4% paraformaldehyde (PFA) to fix the brain. The brain was dissected out and post-fixed overnight in 4% PFA at 4 °C. A vibratome (Leica) was used to cut coronal sections at 40 μm and these sections were stored in 0.1 M PB at 4 °C. For human brain tissue staining, 50-μm sections of 4% PFA-fixed human hippocampus were cut on a freezing microtome. Sections were rinsed three times in phosphate-buffered saline (PBS; 12 min each time) after removal from the storage protection solution. Both mouse and human brain sections were pretreated with blocking solution (0.3% Triton-X and 10% normal donkey and goat serum in 0.1 M PBS) for 2 h, and then incubated for 48 h with the following primary antibodies (in blocking solution at 4 °C): polyclonal anti-GFAP (chicken, 1:1,000, Millipore, AB5541); polyclonal anti-GABA (guinea pig, 1:1,000, Millipore, AB175); polyclonal anti-glutamate (rabbit, 1:300, Abcam, ab9440); polyclonal anti-Glutamate decarboxylase 67 (GAD67, rabbit, 1:100, AnaSpec, 53501); polyclonal anti-GAT3/4 (Abcam, rabbit, 1:100, ab431; and Millipore, rabbit, 1:500, AB1574), both specific for human and rat GAT3 and mouse GAT4); monoclonal anti-GAD65 (Mouse, 1:200, Developmental Studies Hybridoma Bank); polyclonal anti-GABA A -R α5-subunit (rabbit, 1:200, Abcam, ab10098); monoclonal anti-beta amyloid 1–42 (rabbit, 1:2,000, Invitrogen, 700254). After washing three times in PBS with 0.01% triton-X, the brain sections were incubated with appropriate secondary antibodies conjugated to Alexa Fluor 488, Alexa Fluor 546 or Alexa Fluor 647 (1:300, Molecular Probes), FITC or TRITC (1:500, Jackson ImmunoResearch) for 2 h at room temperature. To reveal the location of Aβ plaques, the brain sections were incubated in PBS containing 2 μg ml −1 thioflavin-s for 12 min, followed by washing in PBS for three times (3 × 12 min). To reduce lipofuscin like-autofluorescence in human brain sections, the Autofluorescence Eliminator Reagent (Millipore, 2160) was used, which did not adversely affect other fluorescent labelling in the section. The brain sections were mounted on a glass slide with an antifading mounting solution with or without 4′,6-diamidino-2-phenylindole (Invitrogen). Fluorescent images were obtained with an Olympus confocal microscope (FV1000) and analysed using the Image J software. Hippocampal slice preparation and recording Mice were anaesthetized with 2.5% Avertin. After decapitation, brains were rapidly dissected out and placed in ice-cold cutting solution containing (in mM): 79 NaCl, 80 sucrose, 26 NaHCO 3 , 10 glucose, 2.5 KCl, 1.25 NaH 2 PO 4 , 7 MgSO 4 and 0.5 CaCl 2 for tonic current recordings. The cutting solution for field EPSP recordings contained (in mM): 230 sucrose, 26 NaHCO 3 , 20 glucose, 2.5 KCl, 1.25 NaH 2 PO 4 , 10 MgSO 4 and 0.5 CaCl 2 . Both solutions were bubbled with 95% O 2 /5% CO 2 . Hippocampal slices were cut at 350 μm with a vibratome (VT1200S, Leica, Germany) and transferred to a transitional chamber containing one half cutting solution and one half standard artificial cerebrospinal fluid (ACSF). The ACSF was composed of (in mM): 125 NaCl, 2.5 KCl, 1.3 MgSO 4 , 26 NaHCO 3 , 1.25 NaH 2 PO 4 , 2.0 CaCl 2 and 10 glucose (290–300 mOsm l −1 ; bubbled with 95% O 2 /5% CO 2 , pH~7.4). Slices were then incubated in ACSF at 32 °C for 30 min to recover. Subsequently, slices were maintained at room temperature for another 30 min before recording. Individual slices were then transferred to a submerged recording chamber where they were continuously perfused (2-3 ml min −1 ) with ACSF saturated by 95% O 2 /5% CO 2 at 32 °C. Whole-cell voltage clamp recordings were performed on dentate granule cells using a pipette solution containing (in mM): 135 CsCl, 5 Na-phosphocreatine, 10 HEPES, 5 EGTA, 4 MgATP, 5 QX-314 and 0.5 Na 2 GTP (pH 7.3 adjusted with CsOH, 280–290 mOsm l −1 ). Pipette resistance was 2–5 MΩ, and series resistance was typically 20–40 MΩ. To record tonic GABA current, 10 μM CNQX and 50 μM DL-APV were added into the ACSF to block glutamate receptors. In some experiments, 5 μM GABA was also added into the ACSF to reveal larger tonic GABA current and increase the signal-to-noise ratio. The total tonic GABA current was revealed by the change of holding current after local perfusion of 100 μM BIC (sigma) to block all GABA A -Rs. The tonic current mediated by α5-GABA A -Rs was revealed by local application of 100 nM L-655,708 (Tocris), a selective inverse agonist for α5-GABA A -Rs. The membrane potential was held at −70 mV. Data were acquired using the pClamp 9 software (Molecular Devices; sampled at 10 kHz and filtered at 1 kHz) and analysed with the Clampfit 9.0 software (Molecular Devices). To test neuronal excitability in dentate granule cells, whole-cell current clamp recordings were performed using a pipette solution containing (in mM): 135 K-Gluconate, 10 KCl, 5 Na-phosphocreatine, 10 HEPES, 2 EGTA, 4 MgATP and 0.5 Na 2 GTP (pH 7.3 adjusted with KOH, 280–290 mOsm l −1 ). As dentate granule cells were usually silent under normal condition, we injected appropriate current (~70 pA) to facilitate AP firing at a stable level (~2 Hz) for at least 5 min (serving as control). Then, brain slices were perfused with different drugs for 3–5 min. The AP fire frequency in the last minute of each drug treatment was quantified. Field excitatory postsynaptic potentials were recorded with glass electrodes filled with 1 M NaCl and 25 mM HEPES (pH 7.3) and were evoked every 20 s with a parallel bipolar tungsten electrode (MicroProbes, USA), which was placed at the medial perforant path in the DG. Three evoked responses were averaged to obtain a data point. Stimulation strength was set to a level that produced a field excitatory postsynaptic potential amplitude at ~30% of the maximum response. After stable 20-min baseline recording, LTP was induced by HFS (100 pulses at 100 Hz, three trains in 20-s interval). Y-maze spontaneous alternation task Spontaneous alternation performance was tested as described previously [17] . This learning task does not involve any training, reward or punishment. It allows the assessment of hippocampus-dependent spatial working memory. Each mouse was placed in the centre of a symmetrical Y-maze and was allowed to explore freely through the maze during an 8-min session. The first 2 min were not included for data analysis because mice were exploring new environment. The total number and the sequence of arm entries in the last 6 min were recorded and analysed. Arm entry was defined as the hind paws of the mice had been completely placed in the arm. Analysis was performed in a blind manner. The percentage of alternation is the number of triads containing entries into all three arms divided by the maximum possible alternations (the total number of arms entered−2) × 100. For in vivo i.p. injection of drugs, L-655,708 (1 mg ml −1 ) and SNAP-5114 (50 mM) were dissolved in dimethylsulphoxide and frozen in storage aliquots. The working solution was diluted 10 times in normal saline solution. In order to chronically block the tonic inhibition mediated by α5-GABA A -Rs or astrocytic GABA release through GAT3/4, L-655,708 (1 mg kg −1 ) or SNAP-5114 (50 μmol kg −1 ) or vehicle was injected once every day for 1 week. The last injection was administrated 30 min before behavioural test. BHP assay Three pairs of 6- to 8-month-old WT and 5xFAD littermates were killed with 2.5% Avertin and the brain quickly removed and put into iced-cold PBS to wash out the residual blood. Hippocampi were then dissected out on a cold platform, the wet weight of each sample was recorded, put into autoclaved EP tube and flash-frozen in liquid nitrogen immediately. The samples were stored in a −80° freezer. To make hippocampal homogenate, two freeze-thaw cycles were performed to break the cell membrane before adding 20-μl bath solution per mg tissue into the EP tube. To further fracture the cell, the hippocampal tissue in the EB tube was sonicated for 1 min on ice. The homogenate was centrifuged for 5 min at 5,000 g . The supernatant was then aliquoted and stored at −20° freezer. To test GABA responses evoked by the brain homogenate, HEK293T cells were transfected with α2β3γ2 plasmids and electrophysiology was performed 24–48 h after transfection. A bundle of 3-barrel glass pipette was pulled by a P-97 pipette puller. Before electrophysiological recordings, the stored hippocampal homogenate was further diluted by 100 times in bath solution and then used for puffing experiments. GABA ELISA assay GABA concentration in the mouse hippocampal homogenate was also quantified using mouse GABA ELISA kit (NB-E20434, Novatein Biosciences, Boston, MA, USA), performed according to the manufacturer’s instructions. Data analysis was performed blindly. Hippocampal homogenate was prepared similar to that described above for BHP assay. Data analysis Data were represented as mean±s.e.m. Student’s t -test (paired or unpaired) was used for statistical analysis in two-group comparison. For comparison among multiple groups, one-way or two-way analysis of variance with post hoc tests were used. Statistical significance was set at P <0.05. Behavioural analysis, BHP assay and GABA ELISA analysis were performed blindly. How to cite this article: Wu, Z. et al . Tonic inhibition in dentate gyrus impairs long-term potentiation and memory in an Alzheimer’s disease model. Nat. Commun. 5:4159 doi: 10.1038/ncomms5159 (2014).